Inhomogeneity of the ultrafast insulator-to-metal transition dynamics of VO2 The insulator-metal transition (IMT) of vanadium dioxide (VO 2 ) has remained a long-standing challenge in correlated electron physics since its discovery five decades ago. Most interpretations of experimental observations have implicitly assumed a homogeneous material response. Here we reveal inhomogeneous behaviour of even individual VO 2 microcrystals using pump-probe microscopy and nanoimaging. The timescales of the ultrafast IMT vary from 40±8 fs, that is, shorter than a suggested phonon bottleneck, to 200±20 fs, uncorrelated with crystal size, transition temperature and initial insulating structural phase, with average value similar to results from polycrystalline thin-film studies. In combination with the observed sensitive variations in the thermal nanodomain IMT behaviour, this suggests that the IMT is highly susceptible to local changes in, for example, doping, defects and strain. Our results suggest an electronic mechanism dominating the photoinduced IMT, but also highlight the difficulty to deduce microscopic mechanisms when the true intrinsic material response is yet unclear. Vanadium dioxide (VO 2 ) is one of the prototypical correlated-electron materials, exhibiting an insulator-metal transition (IMT), with a change in resistivity of several orders of magnitude that can be induced thermally at T ∼ 340 K (refs 1 , 2 ), or optically [3] . The photoinduced IMT occurs on subpicosecond timescales, and therefore has a non-thermal basis. This ultrafast transition has been studied using a wide variety of spectroscopies, with short-pulse optical [3] , [4] , [5] , [6] , terahertz [7] , [8] , [9] , X-ray [10] , [11] , [12] and electron diffraction [13] , [14] , [15] techniques. These studies have addressed the ultrafast electron dynamics and lattice structural processes that occur during the transition, in addition to slower behaviour over multi-picosecond to nanosecond timescales. However, the mechanism underlying both the thermal and photoinduced IMT remains unclear. While insulating VO 2 is clearly not a band insulator [16] , the importance of electron correlations and electron–phonon coupling for its properties remain unclear after more than half a century of study, and experimental results conflict with both Mott or Peierls explanations [7] , [16] , [17] , [18] , [19] . For example, degenerate pump-probe studies [5] revealed a limiting transition timescale of 75 fs, suggesting a phonon bottleneck and therefore a structurally limited transition. In contrast, the observation of coherent phonon oscillations above the apparent threshold for triggering the photoinduced phase transition [7] indicates that the photoinduced IMT is decoupled from the structural transition. Much of the work on VO 2 has focused on polycrystalline thin films, grown by a variety of techniques [20] . Recently, differences observed in the ultrafast and thermal properties due to anisotropy and grain size in polycrystalline and epitaxial thin film samples [9] , [21] , [22] , [23] suggest that growth conditions can substantially modify the measured response. These results contributed to the confusion in the interpretation of previous measurements. Furthermore, most spectroscopy techniques average over multiple crystallites, subject to large inhomogeneous strain, which could, for example, create mixtures of different competing phases. While nanoimaging techniques such as scattering scanning near-field optical microscopy ( s -SNOM) [18] can access the heterogeneity in thin films, the complicating extrinsic interactions among crystallites make results difficult to interpret. To overcome the limitations of averaging over ensembles of crystallites and other heterogeneities, we investigate individual VO 2 single microcrystals. We perform degenerate pump-probe microscopy to monitor the femtosecond dynamics following the ultrafast photoexcitation. In addition, we use infrared s -SNOM to probe the nanoscopic details of the evolution of the spatial phase competition in the thermal IMT. These studies allow us to observe the inhomogeneity in the dynamics among the microcrystals measured, finding highly variable timescales associated with the photoinduced bandgap reorganization. In combination with micro-Raman spectroscopy, we systematically study the relationship of crystallographic orientation, insulating phase and temperature to the photoinduced response dynamics. With s -SNOM infrared nanoimaging, we monitor the growth and evolution of metallic and insulating domains through the thermal transition with 10-nm spatial resolution, and find highly temperature sensitive variations in the spatial organization of the domain structure in the individual single crystals. These results suggest a unusually high sensitivity of both the photoinduced and thermal IMT of VO 2 to yet unresolved small perturbations in the form of defects or strain. Single-crystal pump-probe microscopy A schematic of the degenerate pump-probe experiment is shown in Fig. 1a , with details described in the Methods section. We perform frequency-resolved optical gating (FROG) of the laser pulses ( Fig. 1b ) and determine a pulse duration of ∼ 45 fs. We use the pulse characteristics ( Fig. 1c ) as parameters for the fit of the transient reflectivity (see Results section), to resolve 10 s of fs dynamics of the photoinduced transition by deconvolution. 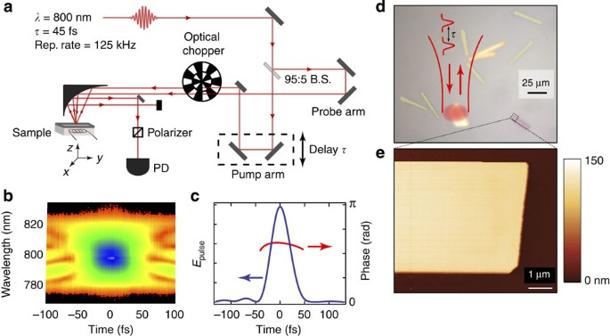Figure 1: Single-crystal VO2ultrafast pump-probe microscopy (a) Schematic of optical layout. (b) Typical FROG spectrogram of pulse, with (c) full phase and amplitude reconstruction in time domain showing∼45 fs pulse duration and small chirp. (d) Optical microscope image of VO2microcrystals on Si/SiO2substrate. (e) Atomic force microscopy topography showing the homogeneous nature of the microcrystals. Figure 1: Single-crystal VO 2 ultrafast pump-probe microscopy ( a ) Schematic of optical layout. ( b ) Typical FROG spectrogram of pulse, with ( c ) full phase and amplitude reconstruction in time domain showing ∼ 45 fs pulse duration and small chirp. ( d ) Optical microscope image of VO 2 microcrystals on Si/SiO 2 substrate. ( e ) Atomic force microscopy topography showing the homogeneous nature of the microcrystals. Full size image The VO 2 microcrystals that we study are grown by vapour transport [24] . They show an abrupt, first-order transition in the absence of strain or doping [25] , in contrast to the percolation behaviour observed in thin-film samples [18] . The crystals vary in size ( Fig. 1d ), and are highly structurally homogeneous, with a flat surface (root mean squared roughness <1.8 nm). We characterize the crystallographic orientation, insulating phase and thermal transition temperature using micro-Raman spectroscopy and s -SNOM [26] for all of the microcrystals measured in these experiments. In the Raman spectra, the shift of the ω V−O Raman mode, at ∼ 600 cm −1 , allows us to estimate the amount of strain within the crystal due to substrate interactions or doping. Three possible insulating structures can be distinguished, monoclinic 1 (M1), intermediate triclinic (T) and monoclinic 2 (M2), with increasing degrees of strain [27] ( Fig. 2a ). With their well-defined, controllable strain state and ability to withstand a high degree of strain, microcrystal samples have been studied to investigate the strain–temperature phase diagrams for VO 2 (see Fig. 2b ) [27] , [28] , [29] , [30] , [31] . The very low-luminescence background and narrow linewidths in Raman spectroscopy indicate a low defect density and confirm a high structural quality of the VO 2 microcrystals. 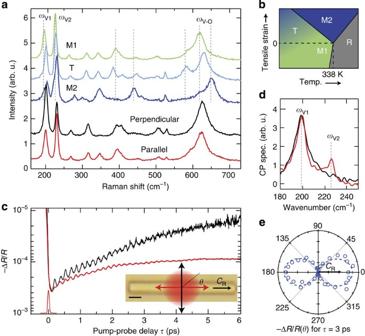Figure 2: Insulating microcrystal phase characterization (a) Raman spectra of the three insulating phases, M1 (green, crystal #1), M2 (dark blue, crystal #20) and intermediate triclinic T (light blue, crystal #4). Perpendicular (black) and parallel (red) Raman polarization with respect tocRof a microcrystal in the M1 phase. (b) Strain–temperature phase diagram showing relation of three insulating phases to metallic rutile phase (gray)27,28. (c) Transient reflectivity traces of crystal #29, −ΔR/R, for low fluence with coherent phonon excitation, with probe polarization parallel (red) and perpendicular (black) to thecRaxis. The pump pulse is shown in red near time zero. Inset: corresponding image of a microcrystal illustrating the probe polarization geometry. Scale bar, 5 μm. (d) Fourier transform spectra of the reflectivity traces, exhibiting phonon modes at∼200 and∼220 cm−1. (e) Reflectivity at 3 ps for different probe polarizations (pump perpendicular to probe). Figure 2: Insulating microcrystal phase characterization ( a ) Raman spectra of the three insulating phases, M1 (green, crystal #1), M2 (dark blue, crystal #20) and intermediate triclinic T (light blue, crystal #4). Perpendicular (black) and parallel (red) Raman polarization with respect to c R of a microcrystal in the M1 phase. ( b ) Strain–temperature phase diagram showing relation of three insulating phases to metallic rutile phase (gray) [27] , [28] . ( c ) Transient reflectivity traces of crystal #29, −Δ R / R , for low fluence with coherent phonon excitation, with probe polarization parallel (red) and perpendicular (black) to the c R axis. The pump pulse is shown in red near time zero. Inset: corresponding image of a microcrystal illustrating the probe polarization geometry. Scale bar, 5 μm. ( d ) Fourier transform spectra of the reflectivity traces, exhibiting phonon modes at ∼ 200 and ∼ 220 cm −1 . ( e ) Reflectivity at 3 ps for different probe polarizations (pump perpendicular to probe). Full size image For low pump fluences, the transient reflectivity response shows an initial electronic excitation, due to the above-gap excitation of the pump, followed by relaxation on a picosecond timescale, as seen in Fig. 2c . Probing at 800 nm (1.55 eV), the response is expected to be dominated by electrons in the d || bands close to the Fermi level [6] , [32] , [33] . The modulations in the reflectivity signal indicate the excitation of coherent phonons in the insulating phase [34] . An orientational anisotropy is evident in the relaxation and coherent phonon behaviour, with faster decay and more prominent oscillations for probe polarization perpendicular (pump parallel) to the crystallographic c R -axis (black line), compared with probe parallel (pump perpendicular; red line). The Fourier transform phonon spectrum, shown in Fig. 2d , reveals an even more pronounced anisotropy. For probe polarization perpendicular to the c R axis, only one low energy phonon peak is resolved, at ∼ 200 cm −1 (6 THz). For parallel probe polarization, both phonon modes emerge, with the second at ∼ 225 cm −1 (6.7 THz). The reflectivity change at 3 ps also shows an angular anisotropy, with a cos 2 θ dependence with angle θ of probe polarization with respect to the c R axis ( Fig. 2e ). At higher fluences, the coherent phonon response is diminished, eventually vanishing for fluences sufficiently high to drive the microcrystal through the photoinduced IMT ( Fig. 3a ). The persistence of the reflectivity change (up to microseconds) indicates a metastable metal-like state. However, without a simultaneous structural probe, we cannot determine the crystallographic structure during this period and whether this state corresponds to a rutile or monoclinic metallic state [19] , [35] , [36] . The inset shows the reflectivity −Δ R / R at 1 ps plotted as a function of fluence, to derive the threshold fluence F th . F th for different microcrystals varies between 2 and 6 mJ cm −2 , which we attribute to variable coupling to the substrate. These values are close to or slightly lower than those observed in thin films, which range from ∼ 5.5 mJ cm −2 up to >15 mJ cm −2 (refs 6 , 11 , 36 , 37 ), due to stronger substrate coupling. 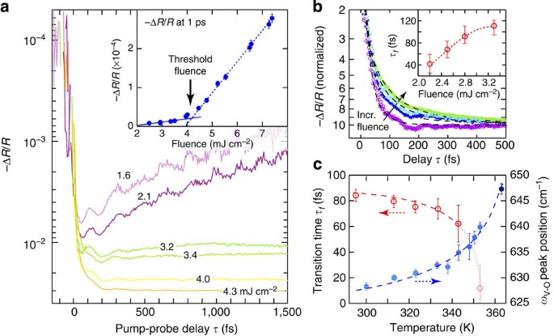Figure 3: Fluence and temperature dependence (a) Fluence-dependent transient reflectivity traces −ΔR/Rfor crystal #30. Inset shows the non-linear dependence of the reflectivity with fluence atτ=+1 ps delay. (b) Change in short timescale dynamics with fluence forF>Fth, on crystal #13. Black lines show fits to exponential recovery behaviour, with extracted transition timeτfshown in the inset. (c) Variation of transition time with temperature, measured at 3.3 mJ cm−2, showing a decrease inτfwith increasing temperature (crystal #30). This is correlated with a change in insulating structure, as monitored through theωV−ORaman mode (seeSupplementary Table 2). Error bars are based on the uncertainties of the fit of equation (1) inτf, and a Lorentzian fit to the V–O phonon Raman line inωV−O. Blue and red dashed lines are guides to the eye. Figure 3: Fluence and temperature dependence ( a ) Fluence-dependent transient reflectivity traces −Δ R / R for crystal #30. Inset shows the non-linear dependence of the reflectivity with fluence at τ =+1 ps delay. ( b ) Change in short timescale dynamics with fluence for F > F th , on crystal #13. Black lines show fits to exponential recovery behaviour, with extracted transition time τ f shown in the inset. ( c ) Variation of transition time with temperature, measured at 3.3 mJ cm −2 , showing a decrease in τ f with increasing temperature (crystal #30). This is correlated with a change in insulating structure, as monitored through the ω V−O Raman mode (see Supplementary Table 2 ). Error bars are based on the uncertainties of the fit of equation (1) in τ f , and a Lorentzian fit to the V–O phonon Raman line in ω V−O . Blue and red dashed lines are guides to the eye. Full size image To quantify the transition dynamics and relate to the physical characteristics of the different microcrystals, we fit the above-threshold transient reflectivity behaviour to . Here f ( t ), the response function of the microcrystal, is convolved with I ( t ), the transient intensity of the pulse from FROG analysis, which accounts for the time resolution and the step-like excitation at t =0 without a priori assumptions about pulse duration or shape (see Methods section for more details on the convolution procedure). f ( t ) is modelled as a biexponential function: with τ f the initial, ultrashort transition time, constrained to <1 ps. τ s captures the longer timescale behaviour, with 2 ps< τ s <10 ps, R ∞ describes the magnitude of the reflectivity change and the parameter a sets the relative scaling of the fast and slow exponential terms. We find that the contribution from slow dynamics is generally small (that is, a <<1) and therefore we focus here on the short timescale dynamics captured by τ f . Representative fits of the transient reflectivity response for crystal #13 for a range of above-threshold fluences are shown in Fig. 3b (black dashed lines), with −Δ R / R normalized for clarity. For the <500-fs range, the response is dominated by τ f . We observe three distinct characteristics in the ultrafast initial response. First, for the lowest fluence investigated we see a transition time of τ f =40±8 fs, shorter than the previously observed dynamics in any VO 2 sample, as discussed further below. Second, we observe a dramatic, up to threefold increase in transition time with increasing fluence (b, inset), in contrast to a decrease observed in previous work on polycrystalline films [3] , [6] . Third, we see the transition time τ f decrease with increasing sample temperature ( Fig. 3c ). During the measurement, we used sufficiently low laser repetition rates (<100 kHz) to allow complete relaxation to the initial insulating state, thus minimizing the effects due to hysteresis that can occur close to the transition temperature. Through the combination with Raman spectroscopy, we can correlate this temperature-dependent change with the structural changes of the insulating phase on heating, as has been observed previously [27] . The pump-probe measurement at T =352 K has a small change in transient reflectivity and large uncertainty, since at this temperature metallic domains have appeared due to thermal excitation. The data shown in Fig. 3 are for two different microcrystals. Figure. 3a,c shows fluence and temperature dependence for crystal #30 (see Supplementary Fig. 1 and Supplementary Note 1 for discussion of hysteresis effects during the thermal MIT transition) and Fig. 3b shows data for crystal #13, respectively. The trends of an increase in τ f with increasing fluence and a decrease in τ f with increasing temperature are seen for all measured microcrystals, though extracted transition times vary between crystals. The transition times τ f obtained from all measurements on 28 microcrystals of different sizes, and for selected different initial temperatures, and range of fluences are summarized in Fig. 4 and Supplementary Table 1 . The values are shown as a function of the measured ω V−O phonon frequency from Raman spectroscopy, as a proxy for the different insulating phases of the crystals (indicated by green–blue colour bar for the M1, T and M2 phases). The error bars are based on the statistical uncertainties of the fit of equation (1) in τ f , and a Lorentzian fit to the V–O phonon Raman line in ω V−O . Different microcrystal widths are indicated by the size of the data symbols (see legend), from <5 μm to >15 μm. The fluences used are all above the threshold fluence for the specific microcrystal, with values indicated using false colour. The values of τ f vary reproducibly from 40 to 200 fs for each crystallite. Notably, the average value of τ f over all microcrystals is found to be with (blue circle). This value is in striking agreement with transition times τ TF from thin-film studies [5] ( Fig. 4b ). 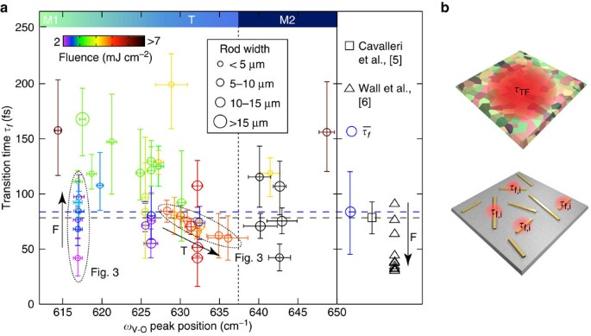Figure 4: Inhomogeneity of the ultrafast IMT (a) Photoinduced transition timeτf, plotted against initial ambient insulating phase, represented by the frequency of the Raman modeωV−O. Error bars are based on the uncertainties of the fit of equation (1) inτf, and a Lorentzian fit to the V–O phonon Raman line inωV−O. Colour bar at top shows corresponding insulating phases. Symbol size reflects microcrystal width, from < 5 μm, to >15 μm. Symbol colour indicates pump fluence, from 2 mJ cm−2(orange) to >7 mJ cm−2(black).τfvaries from∼40 to∼200 fs, with no clear correlation with insulating phase. Dashed ovals indicate data sets shown inFig. 3. Average transition time of all microrod measurements(blue circle/line), compared with (75±15) fs from Cavalleriet al.5(black square/dashed line) observed in thin film samples. Time constants by Wallet al.6from polycrystalline films (525 nm probe wavelength), where a decrease in time constant is observed with increasing fluence, in contrast the behaviour observed here for single crystals. (b) Schematic of thin film (top,τTF) versus single crystal (bottom,τf,i) behaviour. Figure 4: Inhomogeneity of the ultrafast IMT ( a ) Photoinduced transition time τ f , plotted against initial ambient insulating phase, represented by the frequency of the Raman mode ω V−O . Error bars are based on the uncertainties of the fit of equation (1) in τ f , and a Lorentzian fit to the V–O phonon Raman line in ω V−O . Colour bar at top shows corresponding insulating phases. Symbol size reflects microcrystal width, from < 5 μm, to >15 μm. Symbol colour indicates pump fluence, from 2 mJ cm −2 (orange) to >7 mJ cm −2 (black). τ f varies from ∼ 40 to ∼ 200 fs, with no clear correlation with insulating phase. Dashed ovals indicate data sets shown in Fig. 3 . Average transition time of all microrod measurements (blue circle/line), compared with (75±15) fs from Cavalleri et al . [5] (black square/dashed line) observed in thin film samples. Time constants by Wall et al . [6] from polycrystalline films (525 nm probe wavelength), where a decrease in time constant is observed with increasing fluence, in contrast the behaviour observed here for single crystals. ( b ) Schematic of thin film (top, τ TF ) versus single crystal (bottom, τ f,i ) behaviour. Full size image s -SNOM imaging The large variations in τ f indicate that the photoinduced IMT is highly sensitive with respect to unknown electronic or structural heterogeneities between different crystallites. This inhomogeneity appears to be uncorrelated with structure, strain, temperature or microcrystal size, with no consistent behaviour even between crystals attached to the substrate (that is, strained) or free. This suggests a high susceptibility of τ f to minor variations in doping, stoichiometric details or defects. These variations are small enough that they are not reflected in the lattice structure at the level detectable by few-wavenumber Raman shifts, nor in the macroscopic strain or temperature dependence of the IMT. They in turn may be spatially inhomogeneous and lead to spatial variations in the IMT on the intracrystalline level. We take advantage of the complex phase behaviour of microcrystals attached to the substrate, where the minimization of strain to accommodate the different thermal expansions of VO 2 and the silicon substrate leads to the formation of metallic stripe domains along the c R -axis [26] ( Fig. 5 ). These mesoscopic domains with the spatial phase coexistence of metallic and insulating regions provides a sensitive measure to resolve the effect of microscopic inhomogeneities on the thermal IMT, from the interplay of extrinsic strain with localized defects and impurities. 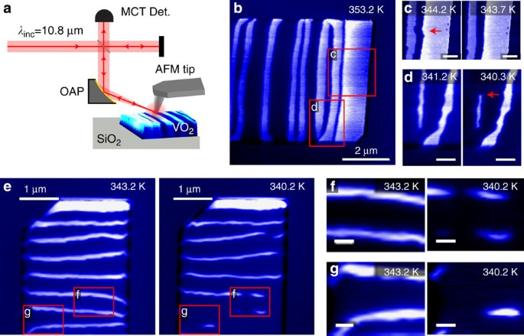Figure 5: Nanoscale inhomogeneity of thermal IMT (a) Schematic of Drude responses-SNOM. (b) When heating through the metal-insulator transition, the microcrystals form alternating metallic (bright) and insulating (dark) domains perpendicular with respect to thecR-axis to minimize substrate strain26. On cooling, the metallic domains gradually narrow and become irregular, eventually breaking into small metallic puddles, with texture sensitive to small variations in temperature (c,d,f,gshow the evolution of corresponding fine structural details). Over repeated cooling cycles, the domains break in different locations and at varying temperatures (seeSupplementary Fig. 2andSupplementary Note 2). The scale bars inb,candf,gare 500 and 200 nm, respectively. Figure 5: Nanoscale inhomogeneity of thermal IMT ( a ) Schematic of Drude response s -SNOM. ( b ) When heating through the metal-insulator transition, the microcrystals form alternating metallic (bright) and insulating (dark) domains perpendicular with respect to the c R -axis to minimize substrate strain [26] . On cooling, the metallic domains gradually narrow and become irregular, eventually breaking into small metallic puddles, with texture sensitive to small variations in temperature ( c , d , f , g show the evolution of corresponding fine structural details). Over repeated cooling cycles, the domains break in different locations and at varying temperatures (see Supplementary Fig. 2 and Supplementary Note 2 ). The scale bars in b , c and f , g are 500 and 200 nm, respectively. Full size image Figure 5a shows a schematic of s -SNOM nano-infrared probing of the Drude dielectric response of VO 2 microcrystals on heating and cooling through the phase transition, with ∼ 10 nm spatial resolution. Figure 5b shows the formation of mesoscopic metallic stripe domains perpendicular to the c R -axis on cooling, with straight domain walls and homogeneous behaviour initially as the insulating states begin to form. Panels c and d then show the gradual narrowing of the metallic domains on further cooling, associated with the emergence of complex, meandering domain walls, with details very sensitive to temperature. The metallic domains then begin to break up in the direction perpendicular to the c R -axis ( Fig. 5e–g ). The domain wall roughening and inhomogeneous disappearance of the metallic puddles on cooling is highly variable with repeated temperature cycling (see Supplementary Fig. 2 ). This nanoscale thermal domain behaviour, with both reproducible and non-reproducible spatial features, together with the variability of the ultrafast IMT dynamics, supports a hypothesis of an electronically driven transition, yet sensitively affected by both static and dynamic variations in the local properties, as discussed further below. In the following, we discuss the implications of the experimental observations of the ultrafast photoinduced IMT dynamics and thermal spatial nanodomain behaviour of single VO 2 microcrystals, especially with regard to the interpretation of previous experiments on polycrystalline thin films. Below threshold, we resolve the dynamical response of the two low-frequency modes in the coherent phonon spectrum, at ∼ 200 and ∼ 225 cm −1 . These modes are of A 1 g symmetry, and are attributed to twisting of vanadium dimers, with their relative strength depending on the type of insulating phase and crystal orientation with respect to pump and probe polarization [34] , [38] . Frequencies and linewidths are consistent with corresponding incoherent Raman scattering and track the different insulating phases, of M1, M2 and triclinic with their characteristic frequencies. Previous coherent phonon measurements have disagreed in whether one or two phonon modes are observed in the 200-cm −1 range (6 THz vicinity), and in their precise frequencies [35] , [39] . These findings can now be reconciled given possible different insulating phases of the crystallites in the thin films. The modes that are observed can depend on both number and relative orientation of the ensemble of crystallites probed in polycrystalline films. Above the fluence threshold for the IMT, we observe ultrafast dynamics on the tens of fs timescale, with a collapse in the bandgap of the insulating phase. In thin film measurements, the fluence-dependent behaviour has been divided into three regimes [6] , [7] : below threshold, where coherent phonons are resolved; above threshold, where the system is driven into the metallic state but thermal effects are visible over longer timescales; and a saturation regime, where the magnitude of the transient reflectivity signal saturates and long timescale thermal behaviour is no longer observed. In contrast, our fluence-dependent measurements on single microcrystals show only two distinct fluence regimes ( Fig. 3 ): the below-threshold regime where coherent phonons are observed and the reflectivity relaxes on picosecond timescales, and the above-threshold regime with emergence of the metastable metallic phase and no long timescale (ps) thermal behaviour. In the saturation regime of thin films, in general, the rapid initial change and persistence of the change in reflectivity indicates that the entire probed volume experiences an ultrafast photoinduced transition to a metal-like state. Since the crystals are thinner than the penetration depth of ∼ 180 nm at 800 nm wavelength, a homogeneous excitation of the microcrystal can be assumed for all above-threshold fluences with the increase in transient reflectivity with increasing fluence attributed to greater excitation density. This is supported by the observation that the microcrystal thickness does not appear to affect transition time. Hence, we conclude that the microcrystal fluence-dependent behaviour differs from the thin films due to its lack of inhomogeneous crystallite contributions, with different threshold fluences, which produce the effective intermediate ‘above-threshold’ regime in thin films. Most notably, we find that the initial insulating phase (M1, M2 or T) has no influence on the dynamics of the ultrafast IMT. Furthermore, crystals with apparently identical lattice structure as concluded from identical Raman spectra reveal different photoinduced transition timescales. This suggests that the emergence of the metallic phase in the photoinduced IMT is not a lattice related effect and the variations in the IMT dynamics point to an electronic delocalization transition. With the transition times observed below the 75-fs half-cycle period of the ω V 1, V 2 phonon modes, the fastest being 40±8 fs, across a range of fluences, we deduce that the 150-fs timescale for breaking the V–V dimer bonds does not pose a rate-limiting step for the formation of the metallic state of the photoinduced transition, as originally proposed by Cavalleri et al . [5] , [15] . Our range of timescales is similar to that reported by Wall et al . [6] shown in Fig. 4 , but their results are not directly comparable since they are based on a model with additional time constants and fitting parameters, and were extracted from dynamics measured at a different probe wavelength. We also note that Wall et al . [6] additionally observed a strong dependence of the dynamics on wavelength. While measurements close to the fluence threshold may contain fast contributions from photoexcited carriers without an associated bandgap collapse, all measurements shown in Fig. 4a show a persistent, long timescale reflectivity change up to microseconds in duration with no subsequent relaxation on the few-ps timescale, indicating an electronic phase change. We also note that very low fluence thresholds for the electronic transition and a monoclinic metallic phase have been proposed recently [36] , [40] , which is consistent with our observations. Our results also suggest a finite response time for the transition [40] . The electronic origin of the dynamics is supported by the decrease in transition time observed on heating the microcrystals. While the free energy change with the increase in temperature is small [41] compared with the energy deposited by the pump pulse, the change in dynamics we observe is substantial. The insulating phase also changes with increasing temperature, following the progression M1–T–M2 (as shown in Fig. 3 ), but the structural change in itself appears to have no effect on the transition time, as discussed above. This temperature-dependent decrease in transition time is an interesting counterpoint to the increase in transition time with increasing fluence. This behaviour is in contrast to Wall et al ., whose time constants all decreased with increasing fluence [6] . Our results support the hypothesis of a possible artifact of thin-film polycrystalline studies, which probe an ensemble averaged response of variable numbers of crystallites, each with varying transition times and threshold fluences. The ensemble measurement will therefore appear to be a superposition of multiple timescales, requiring a larger number of fitting parameters and producing different fluence-dependent behaviour. Fluence behaviours similar to that observed here were previously observed in graphite [42] and Cr-doped V 2 O 3 (ref. 43 ). For VO 2 , this could suggest that the higher fluences drive the system further out of equilibrium and lead to slower transition times to the metallic state. A possible mechanism would be non-equilibrium interband excitations, with variable fractional pump-induced occupation depending on the density of states and its variation with doping and impurities, to states supporting or opposing band structure collapse, as illustrated schematically in Fig. 6a,b . Saturation of states favourable to fast transitions could occur at higher fluences, and would lead to slower dynamics with increasing fluence due to increased excitation of states opposing band structure collapse. The increase in transition time with increasing fluence could also be indicative of a transition driven by an overdamped phonon response, where the damping increases with increasing fluences and leads to slower dynamics. The presence of defects and spatial variations in local doping or strain could furthermore pin domain walls and produce the meandering domain structure we resolve experimentally domain walls ( Fig. 6c,d ). 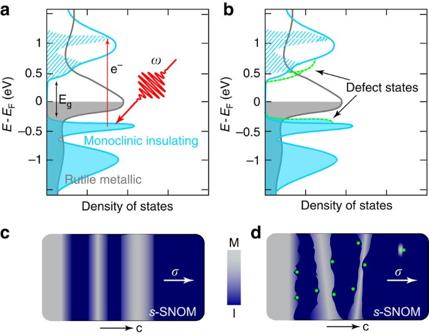Figure 6: Perturbation of the electronic structure and dynamics by defects or impurities (a) Schematic representation showing the electronic band structure of VO2and (b) possible modifications by defects or impurities (green dashed lines), which could modify the transition dynamics of the ultrafast IMT and produce the variable dynamics observed. These defects could also sensitively affect the spatial IMT nanodomain behaviour as observed experimentally (c,d). Figure 6: Perturbation of the electronic structure and dynamics by defects or impurities ( a ) Schematic representation showing the electronic band structure of VO 2 and ( b ) possible modifications by defects or impurities (green dashed lines), which could modify the transition dynamics of the ultrafast IMT and produce the variable dynamics observed. These defects could also sensitively affect the spatial IMT nanodomain behaviour as observed experimentally ( c , d ). Full size image In summary, even on the individual-crystal level for nominally homogeneous single crystals, we observe a highly inhomogeneous IMT behaviour, with dynamics ranging from ∼ 40 to ∼ 200 fs. In addition, s -SNOM imaging of the thermal transition also shows inter- and intracrystal inhomogeneity, with variability of the metallic domains on cooling indicating that the VO 2 microcrystals are in a highly dynamic state close to the critical temperature T C . We therefore conclude that in thin films the intrinsic dynamics can be masked by the inhomogeneous distribution and complicating extrinsic interactions among crystallites. Yet, even on the single-crystal level, both the ultrafast photoinduced studies and thermal IMT s -SNOM indicate a high degree of sensitivity to, for example, dopants and defects. These could alter the density of available states and the redistribution of photoexcited holes and electrons, and thereby change the rate of electron delocalization and subsequent bandgap collapse. Similarly, defects and complex strain could disrupt the free energy uniformity and produce complex domain topology in the thermal transition. Further study of the broadband response of microcrystals could help to elucidate the nature and specific influence of these defects on the mechanism of the IMT. These results raise the question of how to access the intrinsic response of VO 2 , and that of strongly correlated electron materials more generally. Our results call for more precise characterization of VO 2 and other samples, given that the rich and diverse properties of these materials that can be induced and controlled through, e.g., doping, strain, external fields may be more sensitive to disorder and impurities than previously expected. Sample details and Raman characterization The single-crystal vanadium dioxide microcrystals were grown by vapour phase transport on an oxidized silicon substrate [24] . This produces rectangular cross-sectional microcrystals of varying sizes and orientations, as shown in Fig. 1d . Typically, the crystals have widths of 100 nm−15 μm, and lengths up to 1 mm. The rutile c -axis ( c R ) is along the length of the rod. To characterize the individual microcrystals, a home-built Raman microscope with HeNe laser excitation ( λ =632.8 nm) and a 0.8 NA objective (Olympus) is used, with 2 cm −1 spectral resolution. The three insulating structural phases, monoclinic M1, monoclinic M2 and triclinic T, are distinguished principally through the position of the 610–650 cm −1 phonon mode, ω V−O ( Fig. 2a ) [27] . Microcrystals with ω V−O close to 650 cm −1 are in the M2 phase, which can be produced by substrate strain or ∼ 2% Cr doping [26] , [27] . For microcrystals in the M1 phase, ω V−O ∼ 620 cm −1 , and the amount of doping or impurity is < 1% (ref. 44 ). Ultrafast pump-probe microscopy The photoinduced IMT in individual microcrystals is studied by degenerate pump and probe microscopy based on a regenerative amplified Ti:S system (Wyvern, KMLabs), which produces 45 fs pulses at 800 nm ( Fig. 1b ), with a variable repetition rate from 10 to 350 kHz. A 95:5% beamsplitter separates the incident light into the pump and probe arms. The two beams are then recombined with a small spatial offset, passed through a dual-frequency optical chopper, and focused onto the sample using an off-axis parabolic mirror with probe focus size ∼ 15 μm and pump focus size ∼ 30 μm. Variable pump fluences of up to 10s of mJ cm −2 are used. The back-reflected probe, selected by polarization, is detected by a photodiode with lock-in amplification to improve the signal-to-noise ratio. The pump and probe polarizations are orthogonal. FROG is used to characterize the pump and probe pulse transient phase φ ( t ) and amplitude A ( t ). With the intensity profile I ( t )= A ( t ) 2 , we convolute the fitting function in the frequency domain to obtain where f ( t ) is a biexponential function given in equation 1. s -SNOM measurements The samples are mounted on a resistive heater with a thermocouple to enable temperature control within absolute uncertainty ±0.5 K. Atomic force microscopy measurements are used to characterize the heights of the rods chosen for measurements. The rods have rectangular cross-sections with thicknesses of 25–200 nm ( Fig. 1e ). Simultaneous with the atomic force microscopy measurements, we perform s -SNOM with a λ =10.8 μm CO 2 laser source to probe the changes in local reflectivity due to the IMT. How to cite this article: O’Callahan, B. T. et al . Inhomogeneity of the ultrafast insulator-to-metal transition dynamics of VO 2 . Nat. Commun. 6:6849 doi: 10.1038/ncomms7849 (2015).